Competition-driven speciation in cichlid fish Theoretically, competition can initiate divergence in habitat use between individuals of a species, leading to restricted gene flow and eventual speciation. Evidence that sister species differ in habitat use is commonplace and consistent with this mechanism, but empirical experimental support is surprisingly scarce. Here we provide evidence that competition has taken a key role in the evolution of genetically distinct ecomorphs of the Lake Tanganyika cichlid fish Telmatochromis temporalis . Experiments show that differences in substrate use between a large-bodied rock-living ecomorph and a neighbouring small-bodied shell-living ecomorph are mediated by size-dependent competition that drives assortative mate-pair formation. Specifically, adults of the larger ecomorph outcompete adults of the smaller ecomorph on favoured rock substrate, compelling the smaller adults to use shell habitat. These results support a role for competition in maintaining reproductive isolation, and highlight the need to identify ecological processes that impose selection to improve our understanding of speciation and adaptive radiation. The theory of ecological speciation proposes that ecologically based divergent selection leads to the evolution of differences among populations in habitat use, in turn restricting gene flow and promoting reproductive isolation [1] , [2] . Relative success of individual phenotypes on different habitat types will depend on resources available [3] and ecological interactions [4] , [5] (such as competition, predation or parasitism) that impose natural selection upon them. Examples where ecological speciation has been invoked are widespread [6] , [7] and there is abundant phylogenetic and population genetic evidence that the speciation process is frequently associated with divergent patterns of resource use. However, it is often unclear how selection has promoted the divergence of ecomorphs and driven associated assortative mating. There is need for more thorough investigations of how natural selection operates during speciation. Specifically, experimental evidence of competition’s role in speciation has remained elusive [8] , [9] . This is despite the concept being implicit in the work of Darwin [10] , evidence that competition for limited resources can restrict habitat use and geographic overlap of species [11] , [12] , [13] , and signs that competition can drive divergent eco-phenotypic character displacement where closely related lineages occur in sympatry [14] , [15] . Theoretical studies predict competition as a driving force in speciation, particularly in non-allopatric scenarios [16] , [17] . In simulations, competition has either been modelled among individuals in a single environment competing for resource along a single axis (for example, food), or among individuals competing for resources along an environmental gradient (for example temperature, humidity and soil nutrients) [18] , [19] , [20] . Evidence from the resource-use patterns and spatial distributions of sister species pairs in nature conform to expected outcomes of such modelled processes, but direct experimental evidence of competition as a driving force for evolutionary diversification is notably rare. Moreover, whether competition can directly enforce reproduction isolation among populations remains an open question. In this study, we used population genetic and experimental evidence to demonstrate a role for competition in speciation within the cichlid fish adaptive radiation of Lake Tanganyika in East Africa. The littoral shoreline of this lake comprises a mosaic of habitats, alternating between rock, open sand, vegetation-dominated and patchily distributed shell beds [21] , [22] . A species characteristic of the rock and shell habitats is Telmatochromis temporalis (Cichlidae, Lamprologini), a substrate-spawner with biparental care and a lake-wide distribution [23] . To avoid predation by other fishes, mammals or birds, it uses rock or shell substrate for shelter, egg laying and rearing young. It has two distinct ecomorphs, a large-bodied rock-morph (wild adult males: 75.7–88.1 mm standard length (SL), wild adult females: 53.1–62.0 mm SL) and a small-bodied shell-morph (wild adult males: 40.3–44.8 mm SL, wild adult females: 26.8–29.4 mm SL) found on shell beds [23] , which are dominated by empty Neothauma gastropod shells [22] ( Fig. 1a ). The two habitats are typically separated by stretches of sand or muddy habitat [24] , [25] , [26] . Analyses of field-collected samples have shown evidence of reproduction isolation between the T. temporalis ecomorphs [23] , [24] , and has revealed differences between them in reproductive biology (egg number [23] and size at reproduction [23] ) and morphology (body shape [24] ). However, previous research has not identified the mechanisms restricting gene flow, or tested for a genetic basis to observed phenotypic differences. 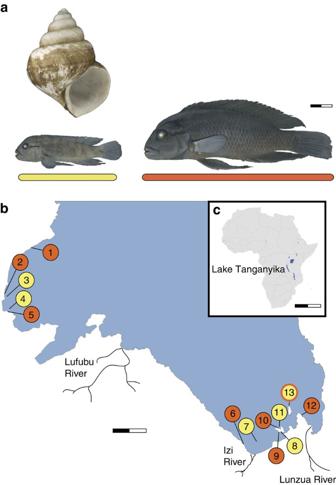Figure 1:T. temporalisfrom Lake Tanganyika. a) The smaller shell ecomorph occupies empty shells of the gastropodN. tanganyicense. Fish pictured are rock (right/orange) and shell (left/yellow) ecomorph males from localities 10 and 11, respectively. Scale bar, 10 mm. (b) Samples for population-level phylogenetic analyses were from 13 sites in the south of the lake. Orange circles=rock habitat sites and yellow circles=shell habitat. Site 13 was mixed rock and shell substrate. Live fish for behavioural experiments were from six sites (2, 3, 4, 5, 10 and 11). Scale bar, 10 km. (c) Map of Africa with the East African Great Lakes, including Lake Tanganyika. Scale bar, 2,000 km. Figure 1: T. temporalis from Lake Tanganyika. a ) The smaller shell ecomorph occupies empty shells of the gastropod N. tanganyicense . Fish pictured are rock (right/orange) and shell (left/yellow) ecomorph males from localities 10 and 11, respectively. Scale bar, 10 mm. ( b ) Samples for population-level phylogenetic analyses were from 13 sites in the south of the lake. Orange circles=rock habitat sites and yellow circles=shell habitat. Site 13 was mixed rock and shell substrate. Live fish for behavioural experiments were from six sites (2, 3, 4, 5, 10 and 11). Scale bar, 10 km. ( c ) Map of Africa with the East African Great Lakes, including Lake Tanganyika. Scale bar, 2,000 km. Full size image Here we present evidence from mitochondrial DNA (mtDNA) sequences and nuclear AFLP (amplified fragment length polymorphism) markers supporting the hypothesis that the shell and rock ecomorphs have diverged due to evolutionary processes operating over local spatial scales. We next demonstrate using a common garden experiment that individuals of the smaller shell ecomorph have greater gonad size than comparably size individuals of larger rock ecomorph. This suggests that differences in development of gonads have a genetic basis, and is consistent with field observations that the shell ecomorph matures at a smaller size than the rock ecomorph [23] , [24] . Finally, we demonstrate using a series of controlled laboratory experiments that divergent habitat-use patterns, and assortative mate-pair formation can be replicated in laboratory conditions, and that habitat use is determined by size-dependent competition for territorial space. Given the widespread evidence for habitat differences between sister species in nature, we conclude that competition may have a broad role in generating patterns of divergent habitat use, which in turn promotes reproductive isolation and eventual speciation. Evolutionary history of populations We sampled 13 populations covering 170 km of shoreline and encompassing both shell and rock habitats ( Fig. 1b ; Supplementary Table 1 ). All shell habitats were in close proximity to rock habitat (range 20 m to 2 km). We reconstructed the evolutionary relationships of sampled populations using mtDNA sequences and nuclear genome-wide AFLP markers ( Fig. 2 , Supplementary Figs 1 and 2 ). 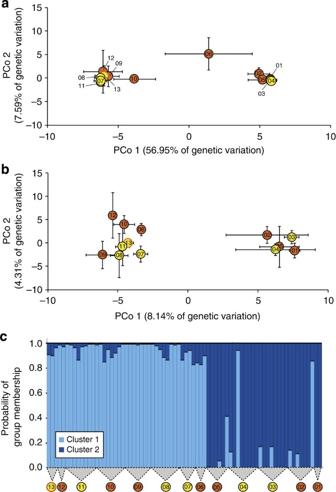Figure 2: Population genetics ofT. temporalis. Principal Coordinate ordination (PCo) of (a) mtDNA (919 bp) and (b) AFLP genetic distances (3,956 loci). Orange circles=rock habitat sites and yellow circles=shell habitat. Numbers within each circle represent sampling sites. Shown are mean values with 95% confidence intervals. (c) Probability of group membership of individuals based on AFLP data, using Structure v.2.3.4 (K=2) dark blue=genetic cluster typical of northern sampling sites; and light blue=genetic cluster typical of southern sampling sites. The results showed that the primary genetic structure was explained by geographic separation among populations, rather than divergence between ecomorphs ( Supplementary Table 2 ). These results imply that the processes that have driven and maintained the phenotypic and genetic divergence between neighbouring ecomorphs occur at the local scale and are consistent with a pattern of parallel evolution, suggested from previous analyses of microsatellite and mtDNA markers [23] , [24] . Figure 2: Population genetics of T. temporalis . Principal Coordinate ordination (PCo) of ( a ) mtDNA (919 bp) and ( b ) AFLP genetic distances (3,956 loci). Orange circles=rock habitat sites and yellow circles=shell habitat. Numbers within each circle represent sampling sites. Shown are mean values with 95% confidence intervals. ( c ) Probability of group membership of individuals based on AFLP data, using Structure v.2.3.4 ( K =2) dark blue=genetic cluster typical of northern sampling sites; and light blue=genetic cluster typical of southern sampling sites. Full size image Common garden analyses of maturation Field studies demonstrate that the shell ecomorph matures at ~25 mm for males and ~20 mm for females, whereas the rock ecomorph matures at ~55 mm for males and ~35 mm for females [23] . 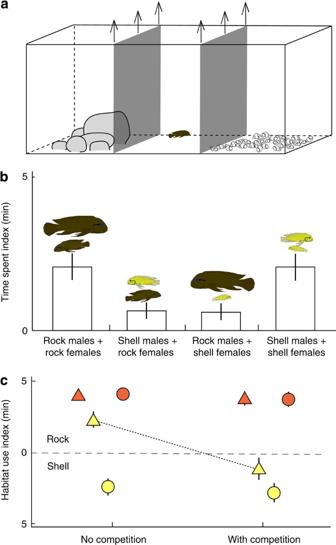Figure 3: Experimental measurements of habitat use and association bias. (a) Setup used to measure habitat use. Shell and rock habitats are separated by sand. Barriers were removed after the fish was introduced, enabling free choice. (b) Test for combined habitat and association choice using a male and female of each ecomorph at the same time (28 trials). Individuals associated assortatively and on their respective habitat. Depicted are means±s.e.m. (c) Habitat use in the absence of a same-sex competitor (no competition); rock males (46 trials); shell males (45 trials); rock females (44 trials), shell females (46 trials) and presence (with competition) of a same-sex competitor; males (28 trials); and females (31 trials). Orange=rock ecomorph, yellow=shell ecomorph, triangles=males and circles=females. Depicted are means±s.e.m. To assess whether these differences have a genetic basis, we quantified gonad mass of two rock-shell population pairs reared in laboratory conditions ( Supplementary Table 3 ). Analyses tested for differences in gonad mass between ecomorphs (rock/shell) and sampling sites (Chibwensolo 2-3, Mbita Island 10-11, Fig. 1 ), while controlling for body mass, in males and females separately. Both sexes of the shell ecomorph had significantly greater gonad mass than equivalents of the rock ecomorph (analysis of covariance (ANCOVA); males F 1,77 =8.714, P =0.004, shell males n =42, rock males n =40; females F 1,84 =26.440, P <0.001, shell females n =43, rock females n =46; Supplementary Fig. 3 ). There was no significant difference between the Chibwensolo or Mbita island sampling sites for males (ANCOVA; F 1,77 =2.667, P =0.106), but a significant difference was present for females (ANCOVA; F 1,84 =4.214, P =0.043). Although the influence of maternal effects cannot be discounted, these results support the hypothesis that life history trait differences observed between the ecomorphs in the natural environment have a genetic basis, and the differences are not exclusively a consequence of phenotypic plasticity. Experiments studying maturation in reciprocal crosses have the potential to further inform us of the genetic basis of the observed differences. Mechanisms driving habitat use and assortative mating To investigate the drivers of divergent habitat use of the ecomorphs, we studied three rock-shell population pairs under experimental conditions ( Fig. 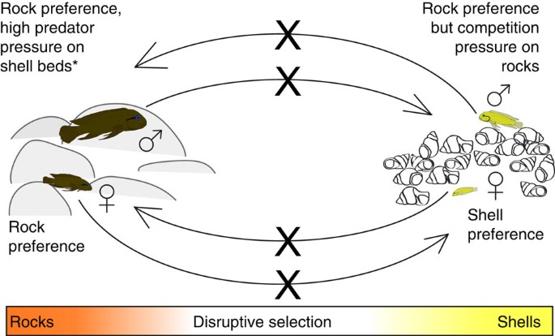Figure 4: Schematic of mechanisms resulting in assortative mating of ecomorphs in adjacent habitats. Arrows indicate potential migration directions between habitats. Crosses indicate factors preventing migration. Asterisk indicates evidence of high predator pressure on rock ecomorphs over shell habitat26. 3a ; Supplementary Table 4 ). In each of these three cases, the adjacent ecomorphs differed significantly from one another in AFLP-based population genetic analyses ( Supplementary Table 5 ). To determine whether the natural pattern of habitat use could be replicated in laboratory conditions, we introduced both a rock and a shell pair (that is, male and female) of individuals simultaneously to an aquarium containing both rock and shell habitat separated by bare sand (Experiment 1, Supplementary Fig. 4a ). During each observation period, we recorded the time individuals spent in association with one another and their time on each substrate. Results showed that there were conspicuous non-random associations of pairs of individuals (analysis of variance (ANOVA); F 3,103 =4.454, P =0.005), with individuals of the same ecomorph associating together significantly more than individuals of different ecomorphs ( post hoc Fisher's least significant difference (LSD) tests P <0.001; Fig. 3b , Supplementary Table 6 ). Moreover, when individuals of the same ecomorph were together, they spent significantly more time on their respective habitat than other habitats (ANOVA; rock ecomorph F 2,81 =27.480, P <0.001; post hoc LSD tests P <0.005; shell ecomorph F 2,81 =13.663, P <0.001; post hoc LSD tests P <0.001; Supplementary Table 6 ). There were no significant effects of collection site-pair on either association bias of individuals or habitat use, suggesting that fish behaved similarly despite originating from different geographic areas ( Supplementary Table 6 ). These data show that the pattern of assortative habitat use and ecomorph pairing observed in the wild can be readily replicated in aquaria. Figure 3: Experimental measurements of habitat use and association bias. ( a ) Setup used to measure habitat use. Shell and rock habitats are separated by sand. Barriers were removed after the fish was introduced, enabling free choice. ( b ) Test for combined habitat and association choice using a male and female of each ecomorph at the same time (28 trials). Individuals associated assortatively and on their respective habitat. Depicted are means±s.e.m. ( c ) Habitat use in the absence of a same-sex competitor (no competition); rock males (46 trials); shell males (45 trials); rock females (44 trials), shell females (46 trials) and presence (with competition) of a same-sex competitor; males (28 trials); and females (31 trials). Orange=rock ecomorph, yellow=shell ecomorph, triangles=males and circles=females. Depicted are means±s.e.m. Full size image We next tested whether individuals were associated with representatives of the same ecomorph, irrespective of habitat using a free choice experimental design where both rock and shell ecomorph stimulus fish of the other sex were presented in jars (Experiment 2, Supplementary Fig. 4b ). We found no patterns of biased association with individuals of same ecomorph in either sex (ANOVA; males F 1,79 =0.980, P =0.324; females F 1,79 =0.735, P =0.394). There was no significant effect of collection site-pair on association behaviour, suggesting that fish behaved similarly despite originating from different geographic areas ( Supplementary Table 7 ). Thus, the hypothesis that the observed ecomorph pairing found in the natural environment is because of direct choice of individuals from the same ecomorph was not supported. We then investigated whether associations between males and females of the same ecomorph observed in the wild are linked to substrate choices by testing for habitat choice in laboratory aquaria. Initially, individual fish were studied in the absence of competitor fish (Experiment 3, Fig. 3c , Supplementary Fig. 4c ). Males from both ecomorphs mostly used rock habitat (ANOVA; rock ecomorph F 1,79 =145.64, P <0.001; shell ecomorph F 1,79 =17.837, P <0.001). Rock ecomorph females used rock habitat (ANOVA; F 1,75 =102.897, P <0.001), and shell ecomorph females used shell habitat (ANOVA; F 1,79 =14.975, P <0.001). There were also no significant effects of collection site-pair on substrate-use behaviour, suggesting that fish behaved similarly despite originating from different geographic areas ( Supplementary Table 8 ). However, habitat use in both sexes was significantly dependent upon SL of individuals (Spearman’s rank correlation: males r s =0.253, n =91, P =0.013; females r s =0.665, n =92, P <0.001; Supplementary Figs 5 and 6 ), suggesting that the primary driver of habitat use may be body size and not necessarily the field-assigned ecomorph to which they belong. We next explored the possibility that large-sized males typical of rock habitat are able to exert a negative competitive influence on smaller males typical of shell habitat. For this, we repeated the habitat-use trials in the presence of a competitor fish of the other morph (Experiment 4, Fig. 3c ; Supplementary Fig. 4d ). We found rock ecomorph males maintained their rock habitat use in the presence of shell ecomorph males (ANOVA; F 1,49 =52.192, P <0.001), but shell ecomorph males lost their rock-use pattern (ANOVA; F 1,49 = 1.730, P =0.1195; Fig. 3c ; Supplementary Fig. 7 ) and shifted significantly towards shell habitat in the presence of rock ecomorph males ( t -test; n 1 =45, n 2 =28, t =3.431, P =0.001). Females maintained habitat-use patterns in the presence of females of the alternative ecomorph (ANOVA; rock females used rock habitat F 1,55 =45.957, P <0.001; shell females used shell habitat F 1,55 =20.802, P <0.001; Fig. 3c ; Supplementary Fig. 7 ). There were significant differences between collection site-pair on habitat use ( Supplementary Table 8 ). Nevertheless, the overall pattern of shell ecomorph males being less likely to use rock in the presence of a rock ecomorph competitor, and more likely to use shell, was observed in all site-pairs ( Supplementary Figs 5 and 7 ). Collectively, these results suggest that the differences between the two ecomorphs have a genetic basis, and that evolutionary divergence has resulted from the action of natural selection on individual habitat use. The population genetic data are consistent with a pattern of genetic isolation by distance, which is not unusual for hard substrate-associated cichlids of the region, and has been shown in other lamprologines ( Variabilichromis moorii [27] and Neolamprologus caudopunctatus [28] ). The population genetic data suggest that the selective processes that have led to diversification have taken place over local spatial scales. The behavioural results support a mechanism where the reciprocal habitat use of the ecomorphs is maintained by ecological interactions and size-dependent habitat-use patterns, rather than direct mate choice ( Fig. 4 ). Specifically, on rock habitat large territorial rock ecomorph males impose ecological selection via competition against small- and intermediate-sized males, preventing them from securing territory and forcing them to use less-favoured shell habitat. Figure 4: Schematic of mechanisms resulting in assortative mating of ecomorphs in adjacent habitats. Arrows indicate potential migration directions between habitats. Crosses indicate factors preventing migration. Asterisk indicates evidence of high predator pressure on rock ecomorphs over shell habitat [26] . Full size image The rapid change in habitat use of shell ecomorph males that we observed in the laboratory experiments can most parsimoniously be interpreted as a direct response to competition for territorial space. It remains to be established whether this is a consequence of exploitation competition, where individuals compete indirectly and passively and for limited resources [29] , [30] , [31] , [32] , [33] , or interference competition, where individuals compete directly often using aggression [34] . It is most parsimonious that interference competition is dominant in this system, as intraspecific territorial control via aggression is well known in cichlids, including lamprologines [35] . Assessment of competitive ability may take place using additional visual, olfactory or auditory cues. It remains a possibility that exploitative competition for limited rock resources has influenced habitat use, and also that the avoidance response of the small ecomorph males has been under positive selection during passive competition for limited resources. We observed size-dependent habitat use in females, with smaller females using shell habitat and larger females using rock habitat ( Fig. 3 ). These apparent preferences may be linked to familiarity of rearing environment that can alter subsequent behaviour in fishes [36] , [37] . However, they could alternatively be an innate behaviour linked to requirements for optimal habitat, and specifically the requirements for self-protection, egg laying and brood care [38] . Small females may be unable to defend shelter on rock habitat because of competition from large growing females, but they may be favoured on shell habitat as they can escape predators and lay eggs deep enough in shells to avoid the numerous egg predators, including freshwater crabs [26] . Similarly, large growing females would be the most successful competitors on rock habitat, and would be favoured by fecundity selection on rock given their higher reproductive potential [26] . However, establishment of mature rock ecomorph females on shell habitat is also likely to be prevented because of the high potential for predation of both adult fish and eggs laid close to shell entrances [26] . Our results suggest that the divergence between shell and rock ecomorphs is maintained by processes that operate locally. Thus, the T. temporalis system is broadly analogous to that of the three-spined sticklebacks where freshwater ecomorphs have undergone parallel evolution from marine ancestors [39] . Theoretically, there are three ways in which functional genetic diversity required for such parallel speciation can be present within a population. Divergence may follow selection on entirely new mutations that evolve simultaneously in allopatric populations. Alternatively, selection could act on the same ancestral polymorphism present in the allopatric populations as standing genetic variation. Finally, the same mutation could evolve in one population, but could be carried to allopatric populations through dispersal and introgression, and then be favoured in all populations by strong selective sweeps. In sticklebacks, it has been argued that repeated evolution is a result of strong selection on standing genetic variation at key functional genes determining freshwater phenotypes [39] . Given the dramatic intraspecific body size polymorphism present in several lamprologines, including Altolamprologus compressiceps and Lamprologus callipterus [25] , it is certainly plausible that standing genetic variation in body size determining loci is an ancestral condition within this lineage. Given the large area and likely persistence of rock habitat during lake-level change relative to the more patchily distributed shell bed habitat, it is plausible that shell ecomorphs evolved from rock ecomorph populations containing ancestral variation for small body size at maturity. We propose a scenario where small maturing phenotypes are outcompeted on rock habitats and associated genetic variants are kept at low frequency. However, when a population is next to a shell bed, which periodically becomes available due to lake-level changes [40] , small maturing fish are able to shift to shell habitat that contains shelter matching their body size, and thus survive and breed assortatively on the novel habitat. This situation could be maintained by dispersal limitation and selective processes. Specifically, territory establishment in both sexes may be driven by competition and predation, and female reproductive output may be driven by egg predation and fecundity selection ( Fig. 4 ). The picture emerging from this study is that a continuous ecological trait, body size, has diverged because of competition and predator-driven natural selection, with resulting size-based habitat-use patterns leading to assortative mate-pair formation between ecomorphs. As these fishes are substrate spawners with biparental care, they require territory before they form pairs, lay eggs and rear young. Although further experimentation is required to identify the factors that influence mate preference in this system, including the sensory modalities and effects of prior experience, our first experiment does provide some insight. It essentially replicated the early stages of this process by allowing the territorial behaviour to establish and mate pairing to begin with fish in closest proximity. Given this breeding behaviour, and evidence that proximity is a reliable predictor of mating decisions in fishes [41] , [42] , [43] , the results allow us to predict that if the egg laying and fry rearing was to occur in competitive conditions, then size-assortative habitat-dependent mating would occur. Moreover, they also allow us to predict that by the removal of competitors we might expect such assortative mating based on habitat and body size to break down. Laboratory experiments with F2 hybrids encompassing the size range observed in the natural environment have potential to test these predictions. There is widespread evidence for intraspecific polymorphisms in habitat use that result in immigrant phenotypes suffering lower fitness and reduced gene flow among ecomorphs [10] , [44] , [45] . Often this habitat divergence is coupled with differences in body size. Large- and small-bodied ecomorphs with different patterns of habitat utilization are present in several prominent examples of ecological speciation, including coregonid whitefishes [46] , sticklebacks [47] and Anolis lizards [48] . This may indicate that size-based competition-mediated habitat use has a broader role in evolution of species boundaries. However, whether speciation is able to complete by this straightforward mechanism alone remains unclear, at least over short timescales and narrow geographic distances. The completion of speciation may additionally require selection to operate on additional phenotype traits that become correlated with observed ecological trait differences [17] , [49] , [50] , [51] . The mechanism we present is, to our knowledge, the first experimental illustration of how competition among populations for territorial space can reduce gene flow and contribute to ecological speciation. In part, the absence of previous demonstrations may be because of difficulty in convincingly demonstrating a direct competitive influence, that ideally should involve experimental manipulations where niche occupancy of individuals is studied in both the presence and absence of competitors [52] . Importantly, our results also indicate that strong sexual selection through direct mate choice is not necessarily required for reproductive isolation to occur between ecomorphs of this species. This does not downweight the importance of evidence for sexual selection by direct choice in speciation of many organisms, including cichlids [53] . It is increasingly plausible that large-scale adaptive radiation results from the combined actions of competition for habitat among populations at carrying capacity, and strong divergent sexual selection, when provided with ecological opportunity [54] . DNA sampling Genetic samples from wild caught T. temporalis were collected from 13 localities in the south of Lake Tanganyika in 2006 and 2010 ( Fig. 1 ; Supplementary Table 1 ). Whole specimens and muscle tissues were collected from 11 populations, and fin tissues were collected only from 2 populations (sites 3 and 4). Samples were preserved in 100% ethanol. DNA extractions were obtained using Qiagen DNeasy Blood & Tissue Kit. mtDNA sequencing The control region (D-loop) was amplified using a newly designed forward primer 5′-ARAGCRYCGGTCTTGTAATCCG-3′ and reverse primer 5′-TGGCTAAATTYACACATGC-3′. Amplified fragments were sequenced using a Big Dye terminator v.1.1 on a 3730xl DNA Analyzer (Applied Biosystems). For the mtDNA population-level analyses an alignment (919 bp) of 163 individuals across 13 populations was generated using Geneious Alignment (default settings) in Geneious 5.6.6 (ref. 55 ). AFLP genotyping DNA for AFLP analysis was extracted from muscle tissue with Qiagen DNeasy Blood & Tissue Kit. Restriction, ligation and pre-amplification was carried out using a LICOR Preparation Kit. For the selective amplification, we used Bioline MyTaq polymerase and 1:10 diluted pre-amplification products. The selective PCR involved three Eco RI primers each labelled with a different fluorescent dye: NED-AAG, FAM-ACA and HEX-ACT and five Mse I primers: 5′-CTGCCACCTCGTCAT-3′. Eco RI primers were combined with every Mse I primers to generate a total of 15 primer combinations. The temperature profile for the selective amplification was as follows: 2 min at 94 °C followed by nine cycles with 30 s at 94 °C, 30 s at annealing temperature, which decreased in each cycle by 1 °C from 66–56 °C, and 2 min at 72 °C. The PCR continued for 20 cycles with 30 s at 94 °C, 30 s at 56 °C, and 2 min at 72 °C, followed by a holding step at 60 °C for 30 min. Selective amplification products were visualized on an ABI3500 Genetic Analyzer (Applied Biosystems) along with an internal size standard (GeneScan-500 ROX, Applied Biosystems). Resulting fragments were automated analysed on Genemapper 4.0. We scored fragments as present with a relative fluorescence unit value threshold of 50. All remaining settings were default. After analysing the samples, we checked fragment/peak calls by eye. Data from samples without clear peak pattern were excluded from final analyses. We used a 96-well plate for samples, extraction repeats, sample repeats and a control. To evaluate the scoring error, all samples were scored twice for three primer combinations. We calculated an error rate of 5.33% for the extraction repeats, 3.70% for sample repeats and 2.74% in scoring repeats. Population genetic structure We first evaluated the evolutionary relationships of all sampled populations using principal coordinate analysis on mtDNA data (single-nucleotide polymorphisms) and genome-wide AFLP marker (presence/absence information) using PAST [56] ( Fig. 2a,b ). We used Structure v.2.3.4 (ref. 57 ) to visualize the probability of group membership of all samples using K =2 to investigate whether the genetic structuring was geographic (north versus south) or between ecomorph (shell versus rock). Each run consisted of 30,000 generations with the first 10,000 as burn-in, and used the recessive alleles model. Without including information of the sampling site, we ran five analyses and found all results to be highly consistent. We therefore present only the result with the highest log-likelihood L ( Fig. 2c ). Analysis of molecular variance [58] in Arlequin v.3.1 (ref. 58 ) was performed separately on the mtDNA and AFLP data, with populations grouped either by sampling region (northern versus southern) or collection habitat (rock versus shell, mixed substrate excluded). Statistical significance was assessed using 10,000 permutations ( Supplementary Table 2 ). mtDNA individual-level phylogenetic analyses A maximum likelihood phylogeny was constructed in RAxML [59] ( Supplementary Fig. 1 ) for D-loop sequence data matrix of 925 base pairs for 164 samples ( Supplementary Table 1 ). The analysis was conducted using the GTR+Γ substitution model and rapid bootstrap values were calculated from 1,000 iterations. mtDNA population genetic differences We focused on the three population pairs used for behavioural experiments ( Supplementary Table 5 ). An alignment of 909 base pairs and 101 individuals from the six populations was generated using Geneious v. 5.6.6. This alignment was used with Arlequin v.3.1 to calculate pairwise distance-based F ST estimator Φ ST , whereas the significance of genetic differences were calculated using a permutation test with 10,000 iterations. AFLP individual-level phylogenetic analyses A neighbour-joining tree ( Supplementary Fig. 2 ) was calculated for the 3,956 characters for 75 samples ( Supplementary Table 1 ) in PAUP* Version 4.0 (ref. 60 ). The optimal criterion was set to ‘Distance’ with all remaining settings set to default. Bootstrap values were evaluated by 1,000 replicates. AFLP population genetic differences We focused on the three population pairs used for behavioural experiments ( Supplementary Table 5 ). This matrix was used with Arlequin v.3.1 to calculate pairwise F ST statistics, and the significance of genetic differences was calculated using permutation tests with 10,000 iterations. Field collections of live fish and husbandry In 2010, wild T. temporalis were collected from three pairs of sites, each pair contained adjacent, but clearly separated populations of rock and shell ecomorphs. Adjacent pairs of sites (referred to as site-pairs) were at Chibwensolo (sites 2 and 3), Ndole/Ntingila (sites 5 and 6) and the north side of Mbita Island (sites 10 and 11) ( Fig. 1 ; Supplementary Table 1 ). Only apparently adult sexual mature individuals were collected. A commercial fish exporter based in Zambia exported collected fish to the United Kingdom. They were kept at the Natural History Museum London, UK. Stock aquaria were kept at a temperature of between 23 °C (winter) and 28 °C (summer), with a 12 h/12 h day/night light rhythm throughout the year. All fish were fed ad libitum with TETRAMIN tropical fish flakes once a day. All behavioural research work was non-invasive and complied with the ethics policy of the Natural History Museum London, UK. Genetic influence on gonad mass at a given body size First generation offspring were reared from fish collected at Chibwensolo (sites 2 and 3) and Mbita Island (sites 10 and 11) ( Fig. 1 ; Supplementary Table 3 ). Several clutches of offspring from each population were pooled into aquaria and reared at an average temperature of 25 °C (seasonal range 23–28 °C), a 12 h/12 h day/night light rhythm and fed ad libitum twice a day with crushed to fine particles TETRAMIN flakes. The number of specimens used for each analysis and their age span are in Supplementary Table 3 . Specimens were killed using an anaesthetic overdose, were fixed in formalin and were washed in water before analysis. The SL of each fish was measured using standard methods [61] with Mitutoyo digital callipers. Individuals were sexed and their somatic mass, ovaries and/or testes were weighed to the nearest 0.1 mg. Behavioural tests of association preference and substrate use All behavioural assays were conducted in 121 × 41 × 55 cm JUWEL Rio aquaria ( Supplementary Fig. 4 ). Before experiments, fish were housed in groups from the same population. Fish SLs were taken with digital calipers to the closest millimetre. No fish was used twice within the same experiment. Sample sizes used in each experiment are provided in Supplementary Table 4 . For all experiments, response fish behaviour was scored using JWATCHER [62] during a 5-min observation time. Experiment 1, combined association preference and substrate use To reconstruct the scenario where both ecomorphs occur on proximate shell and rock habitats, we exposed a pair of rock and shell morphs to one another simultaneously in an aquarium that contained three different substrates ( Supplementary Fig. 4a ). A central section had bare sand, whereas the side sections contained either rock or shell substrate. As rock substrate, we used Atlantic cobbles (12–28 cm diameter) and as shell substrate we used empty Neothauma shells. Fish were introduced and observed as followed. On the morning of day 1, two non-transparent separations were installed, dividing the aquarium into three compartments ( Supplementary Fig. 4a ). A pair of each ecomorph were then released in the middle section of the aquarium. During the afternoon of the same day, the upper part of the separations were removed to enable all fish to explore the substrates and compete for territorial space and substrate. On day 2, the behaviour (for example, time spent where and with whom) was scored for all fish simultaneously during a 5-min observation period using JWATCHER, a key stroke-based software. From the recording files, we initially calculated the time individuals spent in association with one another. However, to ensure that an association bias was being measured, we excluded the time individual fish spent with both ecomorphs of the opposing sex. Thus, we measured the time that: (a) large females were with large males in absence of small males; (b) large females were with small males in absence of large males; (c) small females were with large males in absence of small males; and (d) small females were with small males in absence of large males. Evidence that habitat use of the associating pair deviated significantly from zero was interpreted as a significant habitat bias towards either rock or shell habitat. Four experimental aquaria were used, and the sides of the aquaria containing rocks or shells were randomized. Experiment 2, association preference This experiment aimed to test whether free-swimming individuals favoured associations with stimulus individuals of the opposite sex of their own ecomorph rather than individuals of the other ecomorph. Each experimental aquarium had a 2-cm layer of sand as neutral substrate and was divided into three equally sized sections without separations to allow the response fish to swim freely. The side sections each contained a 2-l clear plastic container, holding the stimulus fish, with an air supply and holes to allow water flow and food intake. The central section was left empty ( Supplementary Fig. 4b ). Fish were introduced, observed and response behaviour was scored after the following protocol. On the morning of day 1, two transparent separations were installed. The stimulus fish (one rock and one shell, individuals of the same sex) were placed into plastic containers ( Supplementary Fig. 4b ). In the afternoon of day 1, the first response fish (of opposite sex to the stimulus fish) was introduced into the central compartment, and 3 h later the separations were removed. On the morning of day 2, the behaviour of the first response fish was observed for a period of 5 min using JWATCHER, and the separations were reinstalled and the first response fish was removed. Next, the second response fish, of a different ecomorph, was released in the afternoon and 3 h later the separation was removed. The behaviour of the second response fish was scored in the morning of day 3 and then all fish were removed. Thus, during each trial two individuals (one of each ecomorph) were exposed to the same stimulus fish. To avoid systematic bias, the order that each ecomorph was used as a response fish was randomized. Similarly, the side of the aquaria where stimulus ecomorphs were placed was changed randomly between trials. We scored and analysed male and female response separately. We used 10 experimental aquaria, with sides of the rock or shell ecomorph stimulus fish randomized between trials. Experiment 3, substrate use with no competition We used the same aquarium setup used in Experiment 1 ( Fig. 3a ; Supplementary Fig. 4c ) to quantify substrate use of individual fish in the absence of competitors. On the morning of day 1, a single fish was released in middle section with transparent separations installed. This separation was removed in the afternoon on the same day. In the morning of day 2, the substrate-use behaviour (time on each substrate) was scored. Fish were introduced, observed and response behaviour was scored as followed. On the morning of day 1, two non-transparent separations were installed, dividing the aquarium into three compartments ( Supplementary Fig. 4c ). An individual fish was then released in the middle section of the aquarium. During the afternoon of the same day, the upper part of the separations were removed to enable the fish to explore the substrates. On day 2, the behaviour (for example, time spent where) was scored during a 5-min observation period using JWATCHER. The time each fish spent on each habitat during the observation period was then calculated. We used 10 experimental aquaria, with the sides of the aquaria containing rocks or shells randomized between trials. Experiment 4, substrate use with competition We used the same aquarium setup as Experiments 1 and 3 ( Supplementary Fig. 4d ) to quantify substrate use of individual fish in the presence of competitors. On the morning of day 1, two fish of the same sex, but from different ecomorphs, were introduced to the central compartment. The upper parts of two non-transparent partitions were removed later the same day, potentially introducing competition for favoured substrate. Fish were introduced and observed, and response behavoir was scored as followed. On the morning of day 1, two non-transparent separations were installed, dividing the aquarium into three compartments ( Supplementary Fig. 4d ). Two fish of the same sex, one of each morph, were then released in the middle section of the aquarium. During the afternoon of the same day, the upper part of the separations were removed to enable the fish to explore the substrates. On day 2, the behaviour of both fish (for example, time spent where) were scored during a 5-min observation period using JWATCHER. The time each fish spent on each habitat during the observation period was then calculated. Four experimental aquaria were used, and the sides of the aquaria containing rocks or shells were randomized. Indices of habitat and association bias From experimental data ‘habitat use’ was calculated as the time fish spent at rocks minus time spent on shells, whereas ‘association bias’ was calculated as the time spent with the rock ecomorph minus the time spent with the shell ecomorph. How to cite this article: Winkelmann, K. et al. Competition-driven speciation in cichlid fish. Nat. Commun. 5:3412 doi: 10.1038/ncomms4412 (2014). Accession codes : The DNA sequences have been deposited in GenBank nucleotide database under accession codes KJ184355 to KJ184518 .